Different types of synchrony in chaotic and cyclic communities Stability and persistence of populations is of great interest for management and conservation purposes. Spatial dynamics can have a crucial role in population stability via synchronization, and beneficial and detrimental effects on population persistence have been shown. Despite a theoretical understanding of synchronization, empirical data on synchrony of populations are restricted to systems that do not display the full spectrum of complex dynamics that may occur in nature (that is, chaos or quasiperiodicity). Here we show in experiments that the qualitative form of dynamic behaviour of chaotic and periodic oscillating communities did not change when unidirectionally coupled to oscillating driver communities. Driver and response populations were phase locked in cyclic communities, whereas chaotic communities showed only short periods of statistical coherencies. Our study provides the first empirical analysis of synchronization of chaotic communities and shows that the likelihood for chaos is not lowered in spatially explicit systems but that cyclic and chaotic systems differ in synchronization. Complex systems can display a variety of dynamics, from steady-state dynamics, to periodic, quasi-periodic or chaotic oscillations. Coupling periodic and chaotic oscillators may cause them to synchronize in different ways [1] , [2] , [3] . As complex nonlinear systems, natural populations exhibit complex, often oscillating dynamics and are generally coupled to other populations, forming spatial structured populations and metapopulations [4] . Synchronization between populations may be caused by migration or dispersal between populations, fluctuating abiotic parameters affecting multiple populations (Moran effect), or trophic interactions with synchronized predators or food resources [5] . Until now, synchronization has been observed for lynx [6] , [7] , voles [8] , measles [9] , [10] , microbes [11] and mussel populations [12] . Synchronization of biological phenomena, such as periodic dynamics of populations, physiological activities or reproductive behavior, have been shown and one principal conclusion of these studies is that synchronization and phase locking can have a fundamental role [11] , [13] , [14] . However, previous studies did not consider more complex dynamics such as chaos and quasiperiodicity that are predicted for complex systems with multi-species interactions as we find them in nature [15] , [16] . The high number of interacting species in nature and the resulting potential of complex dynamics and chaos are of interest, because these complex dynamics are suggested to maintain biodiversity [17] and limit our ability for long-term predictions [18] . Although chaotic dynamics have not been reported for natural populations, there is now accumulating evidence from laboratory studies [18] , [19] , [20] and theory [21] , [22] , [23] , [24] underlining the potential role of chaos. In trying to understand the meaning of chaos for population dynamics, it is necessary to critically evaluate theoretical predictions by manipulative experiments and compare it with systems with cyclic dynamics. Beside in-phase synchronization between spatially separated populations, where populations cycle in tune, a more subtle form, phase locking, has been suggested by ecological models for periodic and chaotically oscillating populations [7] , [11] , [25] , [26] , [27] . Phase locking occurs when one (or more) oscillator influences a second oscillator in such a way that their phases oscillate in tune but that there is a constant difference in the phase of two oscillators [1] , [2] . Phase locking is defined as the locking of the phases of two oscillators and hence the difference between the two phases remains constant, that is, the phase differences Δφ ( t ) = n φ 1( t ) − m φ 2( t ) is constant (φ 1( t ) and φ 2( t ) are the phase of the two oscillators at time t and m , n are integers; in-phase synchronization has zero difference). Phase locking of chaotic dynamics was demonstrated in idealized simple models [28] and observed in laboratory studies of electronic circuits and coupled lasers [29] , [30] but has not been tested experimentally in ecology. Here we test experimentally how cyclic (limit cycles) and chaotic two-prey–one-predator communities synchronize with different driver communities. The relationships between the dynamics of driver and those of the response communities were studied to estimate the effect of synchronization. We used a microbial system in chemostats that has been shown to exhibit a wide range of complex dynamics (steady state, limit cycles and chaos) [19] , [20] , here as a two-stage chemostat system. We found that the qualitative behaviour of chaotic and periodically oscillating populations did not change when unidirectionally coupled to a driver community. However, the results demonstrate clear differences in synchronization between systems differing in their intrinsic dynamical behaviour. For chaotic communities, we found indications for weak degrees of synchronization. In contrast, cyclic communities were phase locked to the driver community. Chemostat system Our two-prey–one-predator systems consisted of the ciliate Tetrahymena pyriformis feeding on the two bacteria Pedobacter sp. and Brevundimonas sp. and steady-state dynamics, limit cycles and chaotic dynamics were established by changing one control parameter. Changes in the dilution rate D of the chemostat system—the fraction of volume that is replaced per day by fresh medium—leads to damped oscillations at D =0.75 d −1 , stable limit cycles at D =0.45 d −1 and chaotic dynamics at D =0.5 d −1 of all three species in single chemostat systems [19] , [20] . We used combinations of two first-stage chemostats with chaotic, cyclic or steady-state dynamics to create different driver communities ( Fig. 1 ). Combining different two first-stage chemostats ( Supplementary Table S1 for the dilution rates and dynamics of the first-stage chemostats and their coupling for the drivers) resulted in driver communities differing in their dynamical behaviour, cycle length and amplitude. Single second-stage chemostats served as response community and were run at dilution rates of D =0.75 d −1 , D =0.5 d −1 , D =0.45 d −1 to create chaotic, cyclic and steady-state dynamics. Response communities received an equal volume from two first-stage chemostats instead of fresh medium. The volume depended on the established dilution rate in the second stage ( Fig. 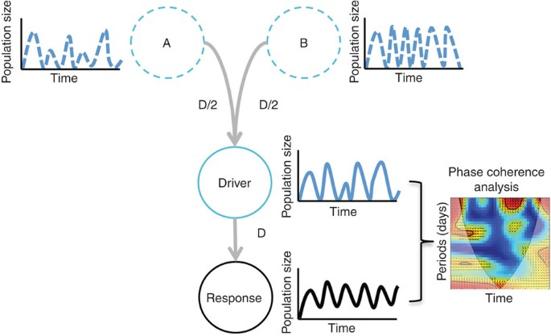Figure 1: Driver–response system used to analyse synchronization of cyclic and chaotic communities. Driver communities were created by continuously mixing communities from two different first-stage chemostats (A and B in the scheme) that had different intrinsic dynamics (steady state, cyclic or chaotic dynamics), here represented by the blue time series with dashed lines. The driver communities (blue time series with solid line) were subsequently pumped into the response community (black time series with solid lines) with a dilution rateD(=migration rate), which was set to D=0.45 d−1for the cyclic andD=0.5 d−1for the chaotic response communities (steady-state dynamics at a dilution rate ofD=0.75 d−1was used as control to see if coupling driver and response introduces additional noise. No effect was observed, seeFig. 2f). The rate by which A and B were mixed was determined by the dilution rateDof the response population. Abundances of the driver communitiesNdriverat time pointtwere calculated byNdriver(t)=NA(t)×D/2+NB(t)×D/2; withNA(t)andNB(t)being the population size in A and B at time pointt, respectively. Driver and response community time series data were then used for phase coherence analysis to detect synchronization. 1 and Table 1 ). Initially, we designed the study to test if response populations in the second-stage chemostat would be entrained by chaotic dynamics in the first-stage chemostats, but there is no evidence for this. Instead, we use the study to test for the synchronization potential for cyclic (limit cycles) and chaotic (irregular) oscillations in the response communities by comparing coherencies of the phase differences between the driver and response communities and populations within a community. We asked the following questions: Do cyclic and chaotic communities synchronize when coupled to a driver community? Are there differences in synchronization between cyclic and chaotic communities? Are phase relations of predator and prey populations within one community changed by synchronization?. Figure 1: Driver–response system used to analyse synchronization of cyclic and chaotic communities. Driver communities were created by continuously mixing communities from two different first-stage chemostats (A and B in the scheme) that had different intrinsic dynamics (steady state, cyclic or chaotic dynamics), here represented by the blue time series with dashed lines. The driver communities (blue time series with solid line) were subsequently pumped into the response community (black time series with solid lines) with a dilution rate D (=migration rate), which was set to D=0.45 d −1 for the cyclic and D =0.5 d −1 for the chaotic response communities (steady-state dynamics at a dilution rate of D =0.75 d −1 was used as control to see if coupling driver and response introduces additional noise. No effect was observed, see Fig. 2f ). The rate by which A and B were mixed was determined by the dilution rate D of the response population. Abundances of the driver communities N driver at time point t were calculated by N driver (t)=N A (t) × D/ 2 +N B (t) × D/ 2; with N A (t) and N B (t) being the population size in A and B at time point t , respectively. Driver and response community time series data were then used for phase coherence analysis to detect synchronization. Full size image Table 1 Dilution rates of response communities and estimated LEs. Full size table Community dynamics We found the response communities and populations in the second-stage chemostats robust in their dynamical behaviours despite the influence of the driver. We saw consistent differences in the dynamical behaviours for the respective dilution rates ( Fig. 2 , black lines). Stable limit cycles ( Fig. 2a ), chaotic dynamics ( Fig. 2c–e ) and steady-state dynamics ( Fig. 2f ) were observed in the response communities. For chemostats showing stable limit cycles, at a dilution rate of D =0.45 d −1 , the estimated Lyapunov exponent (LE) values are close to zero as it is predicted for cyclic dynamics ( Table 1 , Fig. 2a ). Chemostats ran at a dilution rate of D =0.5 d −1 had positive LEs, confirming chaotic dynamics ( Table 1 , Fig. 2c–e ) [19] . The negative LE values for chemostats with a dilution rate of D =0.75 d −1 confirm the observed steady-state dynamics ( Table 1 , Fig. 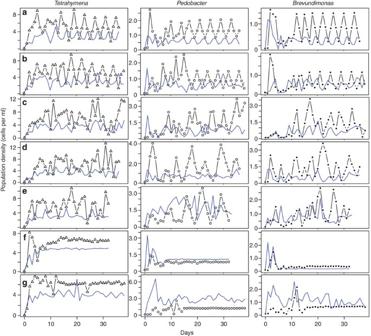Figure 2: Time series data of seven different experimental driver–response systems. Blue lines show densities of the driver (Fig. 1), and black lines and symbols represent densities of the response populations (Fig. 1). Left panels show the dynamics of the predatory ciliateTetrahymena(as 103cells per ml; triangles), middle panels dynamics of the prey bacteriumPedobacter(as 106cells per ml; open circles) and right panel of the prey bacteriumBrevundimonas(as 106cells per ml; filled circles) of the response communities. Chemostats with a dilution rate ofD=0.45 d−1resulted in cyclic communities (a,b), chaotic community dynamics were observed atD=0.5 d−1(c–e) and steady-state dynamics were recorded forD=0.75 d−1(f,g) (Table 1). All data points shown here are the average of three independent samples from each chemostat. 2f ; for a discussion of the use of LEs to quantify the dynamics of experimental time series, see Methods ) Figure 2: Time series data of seven different experimental driver–response systems. Blue lines show densities of the driver ( Fig. 1 ), and black lines and symbols represent densities of the response populations ( Fig. 1 ). Left panels show the dynamics of the predatory ciliate Tetrahymena (as 10 3 cells per ml; triangles), middle panels dynamics of the prey bacterium Pedobacter (as 10 6 cells per ml; open circles) and right panel of the prey bacterium Brevundimonas (as 10 6 cells per ml; filled circles) of the response communities. Chemostats with a dilution rate of D =0.45 d −1 resulted in cyclic communities ( a , b ), chaotic community dynamics were observed at D =0.5 d −1 ( c – e ) and steady-state dynamics were recorded for D =0.75 d −1 ( f , g ) ( Table 1 ). All data points shown here are the average of three independent samples from each chemostat. Full size image Synchronization and phase locking Synchronization and phase locking was determined by examining phase differences between the driver and the response communities in the second-stage chemostats using wavelet coherence analysis and temporal changes of phase differences ( Fig. 1 ; for discussion of the use of this method for short, experimental time series, see Methods ). As a result, we obtained phase coherence plots, which visualize the cross spectrum normalized by the two related auto-spectra as counter plots. Where there is no phase coupling between the driver and the response community, the value is 0 (blue colours in Fig. 3 , Fig. 4 ). For perfect phase coupling, the value is 1 (red colours). Contours (black lines) identify the areas with cross wavelet power spectrum at the 95% power level (coherencies within these contours are significant when tested against red noise). We found that both, cyclic and chaotic communities did not synchronize in-phase with the driver communities (cyclic, Figs 2a ; chaos, Figs 2c–e and 3c–e ), but that synchronization and coherence of the response and driver communities differed between communities displaying cyclic and chaotic dynamics. 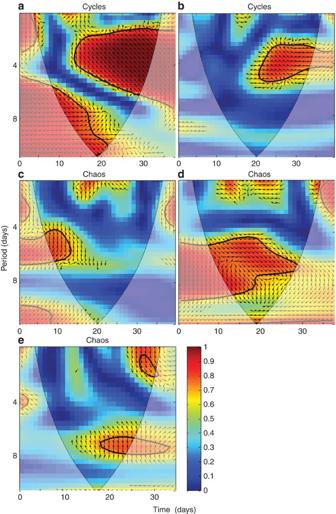Figure 3: Phase relations between driver and response communities in cyclic and chaotic communities. Phase relation of cyclic (a,b) and chaotic (c–e) populations of the preyPedobacterpopulations were analysed using cross wavelet analysis to determine coherences in increase and decrease of the driver and response populations. Results are shown as counter plots (ordinate: time in days; abscissa: common periodicities in the fluctuations of the populations in days) with low wavelet power indicated by blue and high wavelet power by red colours. Black contour lines enclose significant regions in the cross wavelet spectrum and arrows indicate the phase angels between the fluctuations of the driver and response communities. Arrows pointing to the right represents in-phase oscillations (0°) and arrows pointing to the left represent anti-phase oscillations (180°). The shaded areas on both sides of the contour plots represent the cone of influence, where edge effects might distort the signal (for more details on wavelet coherence analysis, seeMethods). Cyclic response communities (a,b) showed clear coherencies with the driver communities (red areas within the significant contour lines) and lagged behind the driver by almost half a period (∼120°; arrows within the contour lines). For chaotic response communities (c–e), there were only short periods of coherencies interrupted by periods without coherencies between the driver and response communities. Similar phase relations were observed for the predatorTetrahymenaand preyBrevundimonaspopulations (Supplementary Figs S1 and S2). The panels correspond to panels inFig. 2. Figure 3: Phase relations between driver and response communities in cyclic and chaotic communities. Phase relation of cyclic ( a , b ) and chaotic ( c – e ) populations of the prey Pedobacter populations were analysed using cross wavelet analysis to determine coherences in increase and decrease of the driver and response populations. Results are shown as counter plots (ordinate: time in days; abscissa: common periodicities in the fluctuations of the populations in days) with low wavelet power indicated by blue and high wavelet power by red colours. Black contour lines enclose significant regions in the cross wavelet spectrum and arrows indicate the phase angels between the fluctuations of the driver and response communities. Arrows pointing to the right represents in-phase oscillations (0°) and arrows pointing to the left represent anti-phase oscillations (180°). The shaded areas on both sides of the contour plots represent the cone of influence, where edge effects might distort the signal (for more details on wavelet coherence analysis, see Methods ). Cyclic response communities ( a , b ) showed clear coherencies with the driver communities (red areas within the significant contour lines) and lagged behind the driver by almost half a period ( ∼ 120°; arrows within the contour lines). For chaotic response communities ( c – e ), there were only short periods of coherencies interrupted by periods without coherencies between the driver and response communities. Similar phase relations were observed for the predator Tetrahymena and prey Brevundimonas populations ( Supplementary Figs S1 and S2 ). The panels correspond to panels in Fig. 2 . 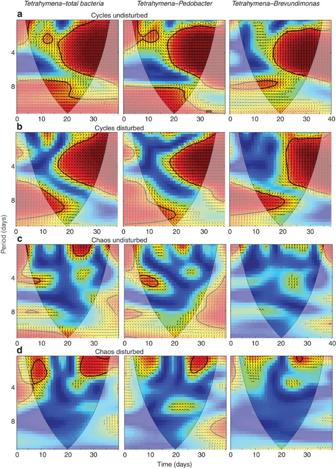Figure 4: Examples of phase relations between populations in cyclic and chaotic communities. PredatorTetrahymenaand total prey (left panels), predatorTetrahymenaandPedobacter(middle panels), predatorTetrahymenaandBrevundimonas(right panels). Statistically significant periodicities are revealed for all cyclic communities for periodic bands between 2 and 4 days (a,b). No differences were observed between undisturbed cyclic communities (a) and cyclic response communities (b). The predatorTetrahymenacycled with a phase lag of a quarter of a period behind the preyBrevundimonas(phase angle∼90°) whileTetrahymenaand the preyPedobactercycled in anti-phase fashion (phase angle∼180°). For chaotic communities, there were no significant relations between the populations within one community (undisturbed,c) and the response communities (d). Data in panelbcorrespond toFigs 2aand3aand, data in paneldtoFigs 2cand3c. For the other communities presented inFigs 2and3, seeSupplementary Figs S5 and S6. Full size image Figure 4: Examples of phase relations between populations in cyclic and chaotic communities. Predator Tetrahymena and total prey (left panels), predator Tetrahymena and Pedobacter (middle panels), predator Tetrahymena and Brevundimonas (right panels). Statistically significant periodicities are revealed for all cyclic communities for periodic bands between 2 and 4 days ( a , b ). No differences were observed between undisturbed cyclic communities ( a ) and cyclic response communities ( b ). The predator Tetrahymena cycled with a phase lag of a quarter of a period behind the prey Brevundimonas (phase angle ∼ 90°) while Tetrahymena and the prey Pedobacter cycled in anti-phase fashion (phase angle ∼ 180°). For chaotic communities, there were no significant relations between the populations within one community (undisturbed, c ) and the response communities ( d ). Data in panel b correspond to Figs 2a and 3a and, data in panel d to Figs 2c and 3c . For the other communities presented in Figs 2 and 3 , see Supplementary Figs S5 and S6 . Full size image For cyclic response communities ( Fig. 2a ), the driver and the response populations fluctuated with a significant periodicity of 2–6 days after the initial transition phase ( Fig. 3a ; red areas). Arrows in the significant regions describing the phase angle between the two communities, point at an average phase angle of ∼ 120°, thus the response communities lagged behind the driver communities by almost half a cycle (that is, almost out-of-phase). Similar results were found for the predator Tetrahymena and the prey Brevundimonas ( Supplementary Figs S1a,b and S2a,b ). For chaotic communities, short periods of synchronization (values close to 1, red colours in Fig. 3c–e and Supplementary Figs S1, S2c–e ) were interrupted by periods with no phase relations between the driver and the response communities (values close to zero, blue colours in Fig. 3 and Supplementary Figs S1 and S2 ). Examinations of the steady-state dynamics in the first and second stage did not reveal externally driven fluctuations or additional noise introduced due to the coupling of the chemostats ( Fig. 2f ). Because wavelet analysis can generically create spurious ‘on’—‘off’ spots (short periods of synchronization interrupted by periods with no significant phase relations) [32] , as we find for the chaotic response communities, we used a second method to examine the relations between the phases of driver and response communities [7] , [33] (see Methods ). Again, we find clear differences between cyclic and chaotic communities. Phase differences in experiments with cyclic response communities were almost constant over time as shown by plateaus ( Supplementary Fig. S3 ) and clear peaks for preferred phase differences in the histograms ( ∼ 0.4; Supplementary Fig. S4 ). Chaotic response communities showed signs of incomplete synchronization with periods where the phase differences were constant (plateaus) and periods with rapid changes indicating phase slips or phase drifts ( Supplementary Figs S3c–e and S4c–e ). The two methods we used to detect synchrony have their limitations when applying to short time series. But both, the phase slips and the short periods of coherence detected by the phase coherence analysis could be indicative for weak degrees of synchronization, such as phase slips and on–off intermittency (see Discussion). Phase relationship between interacting species To gain further understanding into the synchronization behaviour of cyclic and chaotic communities, we analysed the phase relations of the different populations within one community. As a first step, we analysed the phase relations between the predator and the prey populations for cyclic and chaotic dynamics for populations in the first stage of the chemostat system as the undisturbed benchmark using again phase coherence analysis ( Fig. 4a ; Supplementary Figs S5 and S6 ). For cyclic communities, we found a clear band of periodicity between 2 and 7 days for coherence of the predator and the individual prey species and the total prey population after the transition phase ( t ∼1/3 of the period ( Fig. 4a ; Supplementary Fig. S5 left columns) and the Pedobacter prey populations and the predator Tetrahymena cycled in anti-phase fashion, that is, the prey populations reached the maximum density when the predator populations were at lowest densities ( Fig. 4a ; Supplementary Fig. S5 middle columns). Predator and the other prey, Brevundimonas , cycled with a phase shift of a quarter of a period ( Fig. 4a ; Supplementary Fig. S5 right columns). The associations between the dynamics of the populations in the chaotic communities appeared weak and significant only for short time periods ( Fig. 4c ; Supplementary Fig. S6 ). Similarly, predator and prey populations showed no dominant phase relationships. As a next step we looked at the phase relations in the second-stage chemostats with cyclic and chaotic communities ( Fig. 4b ; Supplementary Figs S5 and S6 ) and compared coherence and the phase relations with the undisturbed benchmark of first-stage chemostat communities ( Fig. 4a ; Supplementary Figs S5 and S6 ). For the cyclic communities, clear associations between the dynamics of predator and the two prey populations appeared for periodic bands of 2–7 days, as in the undisturbed communities of the first-stage chemostats. Furthermore, the phase relations between the populations did not change compared with the undisturbed benchmarks. Again, weak or no coherence between the prey and predator populations were detected for dynamics of the chaotic communities. We were able to force cyclical communities to phase lock to the dynamics of a driver community by unidirectional migration, whereas chaotic communities showed only weak degrees of synchronization. To our knowledge, this is the first experimental study, comparing the synchronization behaviour in cyclic and chaotic communities. Previous experimental studies focused on cyclic communities and populations [11] , [34] , [35] . In general, synchronization is considered to arise from dispersal or migration between subpopulations, interactions with a mobile predator or parasite or by spatially correlated environmental variation [5] , [36] . In our experiments, synchronization is predicted to arise solely from migration from one community to another. Synchronization is here not due to the spatial correlation in external parameters or the interaction between external environmental variation and migration (with external entrainment, we would expect to see synchronization in the chaotic communities as well in as in the communities displaying steady-state dynamics). There are two main conclusions to be drawn from this study. First, the character of the oscillations of communities, cyclic or chaotic, did not change when coupled to a driver community, but synchronization differed between cyclic and chaotic communities. Chaotic communities that were subject to migration did not phase lock, although chaos persisted. Instead, we found only short periods where there is phase locking. For the cyclic communities, our study confirms previous observations that migration between cyclic communities can lead to phase-locked dynamics and that the intrinsic cyclical behaviour persists [11] , [12] , [35] , [37] . Interestingly, we did not find the driver and response population cycling in-phase as has been shown in another experimental predator–prey system [11] , instead we found out-phase cycles. The in-phase cycling in the study by Vasseur and Fox [11] was the result of reducing differences in noise at the nadir of a cycle with a net flow from the population with higher densities to the population with lower densities. As a result, the coupled populations emerged from the nadir almost at the same time. This mechanism cannot work in our system because migration is unidirectional and there is no net flow from the population with the higher density to the one with the lower density. This could explain the difference in synchronization (almost anti-phase here, and in-phase in Vasseur and Fox [11] ) between the two systems, but future studies will be needed to test this. Second, the prevalence of chaotic dynamics in the response community was not reduced in comparison to the non-spatial system [19] , [20] and we did not see any sign of dispersal-induced stability as it has been observed for other systems [38] . Spatial structure is often discussed to explain the absence of chaotic dynamics from field records because it might lower the likelihood for chaotic dynamics. For instance, chaos can be suppressed in spatial systems due to the greater impact of noise in spatial systems [39] . Other studies showed that the likelihood for chaotic dynamics is increased in spatially explicit models [40] , [41] , [42] , for example, when dispersal is limited to the lowest trophic level in a three-trophic system [43] . Our system differs from most ecological models for coupled chaotic communities. In our study, migration was unidirectional, corresponding to external or forced synchronization simulating , for example, unidirectional dispersal due to predominating winds or water flow. Almost all the theory on synchronized community and population dynamics in chaotic systems is developed for bidirectional dispersal or as reaction-diffusion model allowing for mutual synchronization [7] , [44] , [45] . One condition for phase locking of forced chaotic systems (that is, unidirectional dispersal) is that the mismatch between the instantaneous phase of the driver and response population is relatively small [46] . Studying the evolution of phase difference between the driver and response communities in our study revealed rapid changes in phase difference between the driver and chaotic response communities ( Supplementary Fig. S3 ), suggesting a large mismatch in the phase between driver and response communities (also seen in Fig. 2c–e ). Strong coupling, as we used in our experiments, of chaotic driver–response systems are predicted to result in in-phase synchronization but unequal coupling between patches or populations might reduce the likelihood of in-phase synchronization compared with systems with equal coupling and migration between the patches [44] , [47] resulting in periods of on–off intermittency [47] , [48] . In our experiment, we saw periods of coherencies and without coherencies supporting this theoretical finding. Phase slips (or phase drifts; Supplementary Figs S4 and S5 ) can also occur close to the boarder of the phase synchronization region and are a transition stage to synchronization of chaotic dynamics [49] . However, we cannot discriminate between patterns such as on–off intermittency as a result of unequal coupling, jumps in phase differences because the system is close to a phase synchronization region or a lack of more accurate analytical tools for short time series [32] . Some caveats are necessary in interpreting our results. Response communities did not only differ in their intrinsic dynamics but also in their migration rates (migration rate: chaos, 0.5 d −1 and cycles, 0.45 d −1 ). Changes in migration rates can affect the synchronization behaviour and the resulting community dynamics [43] . Therefore, it is also possible that the chaotic response populations did not phase lock in the same way as the cyclic response populations because of differences in the migration rate rather than the intrinsic dynamical behaviour. However, differences in migration rates were small and it is unlikely that the differences in synchronization are due to migration rates. Further studies testing explicitly the effect on migration rates on synchronization of chaotic and cyclic systems are needed to clarify this. Second, the recorded time series are short and as discussed above and in the Methods, possibilities to detect chaos and synchrony in such short time series are limited. Nevertheless, there are clear indications that the system behaves chaotically. Most importantly, changes of dilution rates result in different quantitative dynamical behaviours (steady state, limit cycles and chaos) as predicted by a large body of theory [48] , [50] , [51] . This notion in combination with the controlled experimental conditions and the observation that LEs are at least one magnitude larger than the LE values for experiments with limit cycles, suggest that the dynamics are indeed chaotic (although we cannot rule out the possibility of noise-induced oscillations). We used two standard methods for detection of synchrony and both show periods of synchrony and periods without and we conclude weak degrees of synchronization. This observation is supported by theoretical predictions [1] , [2] , [3] , [30] , but as the used methods have limits, we cannot rule out false positives [34] . It is also possible that the quantitative behaviour of the driver community has an effect on synchronization, but the present study does not allow testing for differences. In the case of limit cycles, we see differences in the phase coherence analysis between driver populations that are cyclic ( Fig. 2a ) or irregular ( Fig. 2b ). For the chaotic communities, we found short periods of synchrony in all three response communities independent of differences in the driver dynamics ( Fig. 2c–e ). Further experiments are needed to test for effects of different driver communities. For a better understanding of the different synchronization pattern of cyclic and chaotic communities, we looked if phase relations within one community changed between uncoupled and coupled communities. For chaotic communities, there were no clear phase relations between the prey and the predator population, no matter if the chaotic community was coupled to another community or not. There were consistent phase relations between the predator and the prey populations for cyclic communities but coupling of cyclic communities had no effect on the phase relations between the predator and the prey populations. The predator Tetrahymena and the prey Brevunidimonas cycled in classical consumer resource fashion with the predator lagging a quarter of a period behind the predator, while Pedobacter and Tetrahymena cycled almost in anti-phase fashion. A similar pattern was also found in studies with a similar food web where a predatory rotifer feeds on two genotypes of the same algal species that differ in a trade-off between being defended against grazing and competitiveness [52] , [53] . In the rotifer–algae system, the predator and the less vulnerable prey cycled with a phase shift of more than half a period, the predator lagged behind the more vulnerable prey by a quarter of a period, resulting in almost out-of-phase cycles of the total prey and the predator. Compared with the present bacteria–ciliate system, the phase relation between Brevunidimonas and Tetrahymena (1/4 of a period) suggests that Brevunidimonas is the more vulnerable (preferred) prey. The phase relation of Pedobacter and Tetrahymena ( ∼ 1/2 a period) is similar to the defended prey in the rotifer–algae system, suggesting that Pedobacter is less vulnerable (less preferred) prey. Previous short-term experiments showed a preference of the predator Tetrahymena for one prey species over the other [20] . Tetrahymena ingested four times as many Pedobacter individuals as Brevunidmonas when both prey bacteria were offered at the same density. Thus, we concluded that Pedobacter is the preferred and more vulnerable prey type. It is an open question why the short-term experiments showed the opposite results from long-term dynamics. One possibility is that the predators’ preference changes with frequency or abundances of the two-prey species [54] . Examples for synchronization, both in phase and anti-phase, of cyclic communities in natural systems can be found in literature, although the mechanisms (spatial correlation in external parameters or migration) are not always known [6] , [7] , [8] , [10] , [12] , [55] . Detailed studies on the dynamics of recurrent epidemics suggest that the form of synchronization (in-phase, out-of-phase, anti-phase) depends on the dynamical behaviour, the coupling strength and the dispersal distance [56] . Understanding the mechanisms of spatial synchronization can have important consequences for the dynamics and persistence of metapopulations. In-phase synchronization might be associated with a higher risk of global extinction (for example, after a disturbance) because low population densities occur at the same time in all local populations. Because high and low densities do not occur at the same time in out-of-phase and anti-phase cycling communities, re-colonization from an adjacent population would be possible under these conditions. Weak degrees of synchronization such as on–off intermittency or phase slips could thus be important for maintaining community and species persistence by decorrelation of low minimum population densities in metapopulations. The risk of synchronization and global extinction might be even more reduced for chaotic dynamics because they might show weaker degrees of synchronization in comparison with cyclic communities. With respect to the importance of chaotic dynamics in nature, this is probably one of the best examples of the relevance of chaos in biological systems. Chemostat system Chemostat experiments were performed in a two-stage chemostat systems similar to our previous work [19] , [20] . The two-prey–one-predator systems consisted of the ciliate Tetrahymena pyriformis (CCAP 1630/1 W) feeding on the two bacteria Pedobacter sp. and Brevundimonas sp. (isolated by K. Beck from Lake Schöhsee, Germany). For the one-stage system, changes in the dilution rate D of the chemostat system—the fraction of volume that is replaced per day by fresh medium—lead to damped oscillations at D =0.75 d −1 , stable limit cycles at D =0.45 d −1 and chaotic dynamics at D =0.5 d −1 of all three species [19] , [20] . The second-stage chemostats were coupled to the first stage in such a way, that each second-stage chemostat was connected to two first-stage chemostats. Instead of fresh medium, the second-stage chemostats received an inflow from the two first-stage chemostats they were coupled to (in equal amounts from each first-stage chemostat; Fig. 1 ). Second-stage chemostats were run at dilution rates of D =0.75 d −1 , D =0.5 d −1 , D =0.45 d −1 . All abundances were determined daily [19] , [20] and population densities of the driver populations (inflow to second stage) were calculated from the abundances in the first-stage chemostats and the dilution rate in the second stage ( Fig. 1 ). All experiments were performed at the same time and started from the same inoculums. Data analysis The dynamical behaviour of populations was analysed using calculations of corresponding LE according to the algorithm of Rosenstein [31] , [57] . In general, chaotic dynamics have positive values of one or more of the LEs, systems at steady state have a negative LE and stable limit cycles have values around 0 (should be at least one magnitude smaller than the LE values for chaos and steady-state dynamics). Using the data-driven method by Rosenstein [31] to estimate the LEs allows a direct estimation without further modelling even for short time series. A limit of the Rosenstein method is that we cannot distinguish chaos from noise-induced oscillations. Noise can be introduced by sampling error, demographic and environmental stochasticity, but considering the large population sizes and highly controlled experimental conditions of this study, we argue that the level of noise in our system was relatively low or dampened rapidly. In addition, general models describing two-prey–one-predator systems predict the different observed dynamics—steady state, limit cycles and chaos [50] , [51] . More specifically, simulations with a chemostat model parameterized for Tetrahymena, Pedobacter, Brevunidimonas (used in the present study) reflect the observed experimental dynamics (Groll and Altland (2011), unpublished data). The model correctly predicts doubling of periods into chaos (Roessler attractor) for increasing dilution rates. However, the current model cannot predict the three species steady state at high dilution rates as observed in the experiments. We used wavelet analysis and wavelet coherence measures to study coherence and phase relations between interacting populations under cyclic (limit cycles) and chaotic conditions. Wavelet analysis decomposes local fluctuations observed during a small stretch of time into a series of different frequencies (periods) based on wavelet functions. Wavelet analysis is suitable for analysing time series that contain non-stationary power at different frequencies because a wavelet function captures the local fluctuations in terms of time and frequency [58] . Here we used the Morlet wavelet function. Our empirical time series are short compared with time series usually used for wavelet analysis. Cazelles et al . [59] recommend using time series of 30–40 data points with significant periodic components smaller than 20–25% of the series length. Time series used here have at least 33 data points (with daily sampling) and a cycle length of 4 days, smaller then ∼ 12% of the series length. Wavelet analyses were performed using the MATLAB wavelet coherence package. As an extension to the wavelet analysis, wavelet coherence analysis allows measuring the coherence of fluctuations in two time series. It measures the local correlation between two non-stationary time series at a particular frequency or over a specific period. The value of wavelet coherence, which is the cross spectrum normalized by the two related auto-spectra, falls into the range of 0 and 1. When there is no phase coupling between two time series, the value is 0, and for perfect phase coupling, the value is 1. For further introductions and discussion of wavelet analysis and wavelet coherence for ecological time series, refer refs 58 , 59 , 60 . We used wavelet coherence analysis to study the phase relations of interacting populations within one community, that is, predator and the prey populations, and for measurement of synchronization between coupled communities, that is, the driver communities (inflow) and the response communities in the second-stage chemostats. Results of the wavelet coherence analysis are visualized in contour plots with low wavelet power in the coherence between two time series indicated by blue colours (0) and high wavelet power by red colours (1). Dominant periodic components appear as a horizontal band centred at the periodic components, reflecting the constancy of the periodic components in time. Shaded areas on both sides of the contour plots represent the cone of influence, where edge effects might distort the signal and where the interpretation of the data is limited. Contours (black lines) identify the areas with cross wavelet power spectrum at the 95% power level. Coherencies within these contours are significant (tested against red noise). Arrows describe the phase angle between the populations and obtain information about the sign of the association and the possible phase shifts in the relations. Arrows pointing to the right represent in-phase oscillations (0°) and arrows pointing to the left represent anti-phase oscillations (180°) and a phase lag of half-a-period or cycle. We used a second method to determine synchrony by examining phase differences between the driver and response population. Therefore, we estimated phases for chaotic and periodic dynamics decomposing time series into phase and amplitude by defining quasi-cycles between the maxima (phase increase between the maxima is then exactly 2 π ) and the time dependent phase φ ( t ) is given by linear interpolation [7] . Phase differences between response and driver population were then calculated by Δφ ( t ) =φ 1( t ) −φ 2( t ) , with φ 1( t ) the phase for the response and φ 2 (t) the driver population. How to cite this article: Becks, L. et al . Different types of synchrony in chaotic and cyclic communities. Nat. Commun. 4:1359 doi: 10.1038/ncomms2355 (2013).